A β-synuclein mutation linked to dementia produces neurodegeneration when expressed in mouse brain The discovery of α-synuclein (αS) mutations has made a major contribution to the understanding of the pathogenesis of α-synucleinopathies such as Parkinson's disease and dementia with Lewy bodies (DLB). In contrast, less attention has been paid to β-synuclein (βS) mutations. In this paper, we show that transgenic (tg) mice expressing DLB-linked P123H βS develop progressive neurodegeneration, as characterized by axonal swelling, astrogliosis and behavioural abnormalities, with memory disorder being more prominent than motor deficits. Furthermore, cross-breeding of P123H βS tg mice with αS tg mice, but not with αS knockout mice, greatly enhanced neurodegeneration phenotypes. These results suggest that P123H βS is pathogenic and cooperates with pathogenic αS to stimulate neurodegeneration in mouse brain, indicating a causative role of P123H βS in familial DLB. Given the neuritic pathology of βS in sporadic α-synucleinopathies, it appears that alteration of βS can contribute to the pathogenesis of a broad range of α-synucleinopathies. β-Synuclein (βS) is an abundant pre-synaptic phosphoprotein that is found in the brain and is homologous to α-synuclein (αS) [1] , [2] . Both proteins have been characterized on the basis of their native unfolded structures, but βS is distinct from αS in that βS lacks the majority of the hydrophobic non-amyloid-β component of the Alzheimer's disease amyloid region [3] , [4] . Because of the presence of this highly amyloidogenic non-amyloid-β component, αS is prone to self-aggregate and form toxic protofibrils, whereas βS is less prone to form insoluble aggregates [5] , [6] , [7] . Several lines of evidence suggest that βS may have a protective role against α-synucleinopathies. In support of this notion, overexpression of βS in αS transgenic (tg) mice by either crossing with βS tg mice or using virus-mediated transfer results in amelioration of neuropathology (such as formation of Lewy body-like inclusions) and motor function deficits [7] , [8] , [9] . Mechanistically, βS may directly inhibit aggregation and protofibrillar formation of αS, as demonstrated under cell-free conditions [7] , [10] , [11] . An alternative mechanism may include a role of lipids, as it has been shown that oligomerization of αS is dramatically enhanced by increasing the cellular levels of polyunsaturated fatty acids [12] , which was inhibited by polyunsaturated fatty acid-associated βS in mesencephalic cells [13] . In this context, it is of note that two missense mutations of βS, P123H and V70M, have been linked to familial and sporadic dementia with Lewy bodies (DLBs), respectively [14] . It is possible that the DLB-linked βS mutants might have lost protective functions against the neurotoxicity caused by αS [14] . However, given the autosomal dominant trait of patients with the P123H mutation [14] , toxic gains of function of βS through gene mutation might contribute to the pathogenesis of familial DLB. In support of the latter possibility, our recent study showed that both P123H- and V70M-recombinant βS proteins were prone to aggregate in vitro and that expression of these mutant βS proteins in neuroblastoma cells resulted in lysosomal pathology associated with protein aggregation [15] , [16] . Although DLB is the second most common cause of dementia after Alzheimer's disease [17] , the pathogenic mechanism of DLB is poorly understood. Elucidation of the mechanism through which DLB-linked βS mutations cause neurodegeneration in vivo may provide us with some insights into this critical issue. Accordingly, the main objective of this study was to investigate the neuropathology of DLB-linked P123H βS through analysis of tg mice. The results show that tg mice expressing P123H βS were characterized by neuritic pathology, associated with astrogliosis and behavioural abnormalities. Furthermore, the neuropathology of P123H βS tg mice was not significantly affected by cross-breeding with αS knockout (KO) mice. On the other hand, cross-breeding of P123H βS tg mice with αS tg mice resulted in enhanced phenotypes, including neuronal cell loss and dopaminergic dysfunction. These results strongly suggest that P123H βS is by itself pathogenic and cooperates with pathogenic αS to stimulate neurodegeneration. Neuropathological characterization of P123H βS tg mice We generated tg mice overexpressing P123H βS under the control of the Thy-1 promoter ( Fig. 1a,b ). In all lines of tg mice with P123H βS mRNA expression in the brain ( Fig. 1c ), P123H βS expression was also detected at the protein level ( Fig. 1d ). Mice from line C had the highest levels of transgene expression, followed by the two intermediate expressers, lines B and G, and the three low expressers, lines A, D and E. Lines C and B were analysed in the majority of experiments. 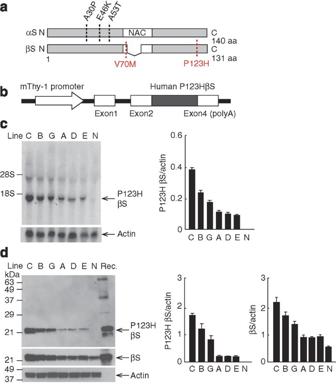Figure 1: Generation of P123H βS tg mice. (a) Scheme shows missense mutations of αS and βS identified in α-synucleinopathies. Two αS mutations, A30P45and A53T46, were discovered in PD, and another αS mutation, E46K47, was later found in DLB. As for βS, two mutations, V70M and P123H, have been reported in DLB14. (b) Diagrammatic representation of the Thy-1–P123H βS construct. (c) Northern blot analysis of P123H βS mRNA. Total RNA (10 μg) prepared from P123H βS tg (lines C, B, G, A, D and E) and non-tg (N) mice brains at 4 months was analysed by northern blotting using32P-labelled P123H βS cDNA (upper panel). The filters were reprobed with32P-actin cDNA (lower panel). Representative blots and data quantified against actin bands are shown as the mean±s.e.m. (n=3). Endogenous mouse βS mRNA was hardly detected with human P123H βS cDNA probe under the current experimental conditions. (d) Immunoblot analysis of P123H βS protein. Total brain extracts (10 μg) prepared from P123H βS tg (lines C, B, G, A, D and E) and non-tg (N) mice at 4 months were analysed using anti-P123H βS antibody, which recognizes P123H βS but not mouse wt βS (upper panel) (Supplementary Table S2). The blots were reprobed with anti-βS antibody, which recognizes both P123H βS and mouse wt βS (middle panel) and anti-actin antibody (lower panel). Recombinant P123H βS (Rec.)15was used as positive control. Representative blots and data quantified against actin bands are shown as the mean±s.e.m. (n=3). NAC, non-amyloid-β component. Figure 1: Generation of P123H βS tg mice. ( a ) Scheme shows missense mutations of αS and βS identified in α-synucleinopathies. Two αS mutations, A30P [45] and A53T [46] , were discovered in PD, and another αS mutation, E46K [47] , was later found in DLB. As for βS, two mutations, V70M and P123H, have been reported in DLB [14] . ( b ) Diagrammatic representation of the Thy-1–P123H βS construct. ( c ) Northern blot analysis of P123H βS mRNA. Total RNA (10 μg) prepared from P123H βS tg (lines C, B, G, A, D and E) and non-tg (N) mice brains at 4 months was analysed by northern blotting using 32 P-labelled P123H βS cDNA (upper panel). The filters were reprobed with 32 P-actin cDNA (lower panel). Representative blots and data quantified against actin bands are shown as the mean±s.e.m. ( n =3). Endogenous mouse βS mRNA was hardly detected with human P123H βS cDNA probe under the current experimental conditions. ( d ) Immunoblot analysis of P123H βS protein. Total brain extracts (10 μg) prepared from P123H βS tg (lines C, B, G, A, D and E) and non-tg (N) mice at 4 months were analysed using anti-P123H βS antibody, which recognizes P123H βS but not mouse wt βS (upper panel) ( Supplementary Table S2 ). The blots were reprobed with anti-βS antibody, which recognizes both P123H βS and mouse wt βS (middle panel) and anti-actin antibody (lower panel). Recombinant P123H βS (Rec.) [15] was used as positive control. Representative blots and data quantified against actin bands are shown as the mean±s.e.m. ( n =3). NAC, non-amyloid-β component. Full size image Histopathological analyses revealed that P123H βS mice are characterized by extensive neuritic pathology. For instance, P123H βS accumulated in various brain regions as early as 6 months of age, including in apical dendrites in the cortex and in axonal deposits in the hippocampus ( Fig. 2a ). Given the lack of βS immunoreactivity for Lewy bodies formed in the autopsy brain with P123H βS mutation [14] 14, it was not unexpected that Lewy body-like inclusions were not observed in P123H βS tg mice. However, one prominent feature of these mice was the formation of P123H βS-immunoreactive axonal swellings in the striatum and globus pallidus ( Fig. 2b ). The number of swellings was well correlated with the expression level of P123H βS and was observed in an age-dependent manner ( Fig. 2b ). Consistent with an abnormal accumulation of P123H βS, the same regions were accompanied by massive gliosis, as revealed by an increased level of glial fibrillary acidic protein (GFAP)-positive astroglia ( Supplementary Fig. S1a–c ). In contrast to P123H βS mice, neither abnormal immunostaining of P123H βS nor gliosis was observed in both non-tg littermates and mice overexpressing wild-type (wt) βS ( Fig. 2a–c , Supplementary Fig. S1a–c ). 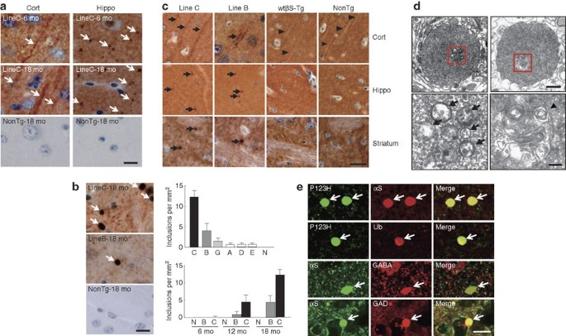Figure 2: P123H βS tg mice are characterized by a neuritic pathology. (a,b) Immunohistochemistry of P123H βS using anti-P123H βS antibody. Ina, P123H βS accumulated in apical dendrites in the cortex (cort, left panels) and in axonal dots in the hippocampus (hippo, right panels) (6 and 18 months (mo)) of P123H βS tg mice (line C, arrows), but not in the same regions of non-tg littermates (NonTg). Scale bar=10 μm. (b) Globules were observed in the striatum and globus pallidus of 18-month-old P123H βS tg mice (lines B and C, arrows), but not in non-tg littermates. Scale bar=10 μm. For quantification, five images were analysed for each mouse and the results were used to calculate the average number of globules per mm2. Upper panel: multiple lines C, B, G, A, D and E, and non-tg (N) at 18 months; lower panel: lines B, C and N at 6, 12 and 18 months. Data are shown as the mean±s.e.m. (n=7). (c) Immunohistochemistry of total βS using anti-βS antibody. βS accumulated in apical dendrites in the cortex (cort), and in axonal dots in the hippocampus (hippo) of 18-month-old P123H βS mice (lines C and B, arrows), but not in wt βS tg mice (wt βS-Tg) and non-tg littermates (NonTg). Arrowheads indicate negative staining of βS in apical dendrites. Similarly, formation of globules in the striatum was observed in 18-month-old P123H βS mice (arrows), but not in age-matched wt βS tg mice and non-tg mice. Scale bar=20 μm. (d) Photomicrographs of two representative globules in 18-month-old tg mice (line C). The lower two panels are insets from the two higher panels. Globules were composed of small vesicles and contained multivesicular bodies (arrows) and autophagosome-like multiple-layered membranous structures (arrowheads). Scale bar=1 μm (upper panel) and 200 nm (lower panel). (e) Anti-P123H βS-immunopositive globules formed in the basal ganglia of P123H βS tg mice (line C, 18 months) were double stained with either anti-αS or anti-ubiquitin (Ub) (upper six panels). Alternatively, anti-αS-immunopositive globules were stained with anti-αS and either anti-GABA or anti-glutamic acid decarboxylase (anti-GAD) (lower six panels). The slides were observed by laser scanning confocal microscopy. Arrows point to globules. Scale bar=10 μm. Figure 2: P123H βS tg mice are characterized by a neuritic pathology. ( a , b ) Immunohistochemistry of P123H βS using anti-P123H βS antibody. In a , P123H βS accumulated in apical dendrites in the cortex (cort, left panels) and in axonal dots in the hippocampus (hippo, right panels) (6 and 18 months (mo)) of P123H βS tg mice (line C, arrows), but not in the same regions of non-tg littermates (NonTg). Scale bar=10 μm. ( b ) Globules were observed in the striatum and globus pallidus of 18-month-old P123H βS tg mice (lines B and C, arrows), but not in non-tg littermates. Scale bar=10 μm. For quantification, five images were analysed for each mouse and the results were used to calculate the average number of globules per mm 2 . Upper panel: multiple lines C, B, G, A, D and E, and non-tg (N) at 18 months; lower panel: lines B, C and N at 6, 12 and 18 months. Data are shown as the mean±s.e.m. ( n =7). ( c ) Immunohistochemistry of total βS using anti-βS antibody. βS accumulated in apical dendrites in the cortex (cort), and in axonal dots in the hippocampus (hippo) of 18-month-old P123H βS mice (lines C and B, arrows), but not in wt βS tg mice (wt βS-Tg) and non-tg littermates (NonTg). Arrowheads indicate negative staining of βS in apical dendrites. Similarly, formation of globules in the striatum was observed in 18-month-old P123H βS mice (arrows), but not in age-matched wt βS tg mice and non-tg mice. Scale bar=20 μm. ( d ) Photomicrographs of two representative globules in 18-month-old tg mice (line C). The lower two panels are insets from the two higher panels. Globules were composed of small vesicles and contained multivesicular bodies (arrows) and autophagosome-like multiple-layered membranous structures (arrowheads). Scale bar=1 μm (upper panel) and 200 nm (lower panel). ( e ) Anti-P123H βS-immunopositive globules formed in the basal ganglia of P123H βS tg mice (line C, 18 months) were double stained with either anti-αS or anti-ubiquitin (Ub) (upper six panels). Alternatively, anti-αS-immunopositive globules were stained with anti-αS and either anti-GABA or anti-glutamic acid decarboxylase (anti-GAD) (lower six panels). The slides were observed by laser scanning confocal microscopy. Arrows point to globules. Scale bar=10 μm. Full size image Electron microscopy (EM) revealed that the swellings were 'globules': small spheroids that are frequently associated with axonal dystrophy ( Fig. 2d ) [18] , [19] . The globules were composed of small vesicles and frequently contained membranous elements such as multivesicular bodies and multilayered membranes. Furthermore, the globules were surrounded by a single membrane with association of no myelin sheaths and no post-synaptic contacts, suggesting that these globules are not functional terminals. Moreover, LC3-positive dots were observed in the globules with an increased amount of LC3-II, a marker of autophagosomes [20] ( Supplementary Fig. S1d,e ). Because cathepsins B and D activities, but not proteasome activities, were significantly decreased in P123H βS tg mice compared with non-tg littermates ( Supplementary Fig. S1f–i ), it is probable that autophagosomes might accumulate in the globules because of decreased clearance by lysosomes. Notably, double immunofluorescence study showed that the P123H βS-positive globules were highly immunoreactive with anti-αS ( ∼ 100%) and to a lesser extent with anti-ubiquitin ( ∼ 70%) ( Fig. 2e ), indicating that endogenous αS and ubiquitinated proteins accumulated because of compromised degradation at the lysosome. A further study revealed that P123H βS-positive globules were also immunostained with both anti-γ-aminobutyric acid (anti-GABA) and antiglutamic acid decarboxylase antibodies ( ∼ 100%; Fig. 2e ). Although few GABAergic neurotransmitters in the basal ganglia, such as dynorphin, enkephalin and substance P, were detected in the globules, a weak immunoreactivity of calbindin was consistently detected ( Supplementary Fig. S2 ), suggesting that the globules were formed in projection-type GABAergic neurons. Because synaptic markers such as synaptophysin and synapsin I and axonal markers including neurofilaments were not detectable ( Supplementary Fig. S2 ), the results suggest again that these GABAergic neuronal terminals are no longer functional. Degeneration of these neurons by P123H βS may be important, as there is ample evidence showing that GABAergic neurons in the striatum, which functions as the second component of the Parkinsonian circuit, are significantly altered in Parkinson's disease (PD) brains [21] . Consistent with the histopathological changes, biochemical analyses showed that expression of P123H βS was increased in an age-dependent manner, particularly in formic acid (FA) fractions, indicating a gradual accumulation of insoluble P123H βS ( Supplementary Fig. S3a ). Compared with P123H βS tg mice, no accumulation of wt βS was observed in FA fractions of wt βS tg mice ( Supplementary Fig. S3b ). Furthermore, upregulation of heat-shock proteins (HSPs), including HSP70 and HSP25, was already apparent at 6 months, whereas expression of synaptic markers, such as SNAP25 and VAMP2, were decreased at 18 months, suggesting that the protective capacity in P123H βS tg mice might be insufficient at this age ( Supplementary Fig. S3c ). Finally, P123H βS tg mice exhibited various types of abnormal behaviours. To determine the effects of P123H βS accumulation on spatial learning and memory, a water maze test was conducted ( Fig. 3 ). In the training sessions, P123H βS mice showed significant learning deficits, whereas non-tg controls performed normally ( Fig. 3a ). Furthermore, P123H βS mice showed significantly less preference for the target quadrant than non-tg littermates, suggesting impaired retention of spatial memory ( Fig. 3b,c ). During the same stage, a home cage test demonstrated that various spontaneous activities were decreased in P123H βS tg mice (line C) compared with non-tg littermates ( Fig. 3d ). In contrast, a rotarod treadmill test showed that motor deficits were not observed in the middle stage (6 months) but became apparent during the late stage (12–18 months) in P123H βS tg mice ( Fig. 3e ). 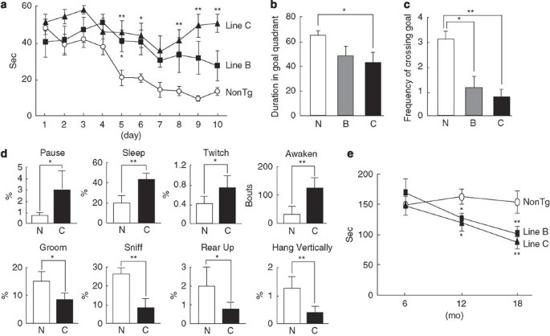Figure 3: Behavioural abnormalities of P123H βS tg mice. (a–c) The Morris water maze test. Compared with non-tg littermates (NonTg), P123H βS tg mice (lines B and C) at 6 months (mo) did not show an improvement in performance during the training session (a). After removing the platform, a probe test was performed on the last day of the training session (b,c). P123H βS tg mice spent less time searching in the target quadrant than did non-Tg (N) mice (b). Similarly, P123H βS tg mice had less frequency of crossing the goal (c). Data are shown as the mean±s.e.m. (n=7–11). *P<0.05, **P<0.01 versus non-tg mice. (d) Home cage test showing decreased spontaneous activities in P123H βS tg mice (line C) compared with non-tg littermates at 6 months. Time spent in various types of behaviours, including 'Pause' 'Sleep' 'Twitch', 'Groom', 'Sniff', 'Rear up' and 'Hang Vertically', was measured using a video tracking system. 'Awaken' is the end of sleep during this period. Data are shown as mean±s.e.m. (n=7). *P<0.05, **P<0.01 versus non-tg mice. (e) The rotarod treadmill test showing impaired motor performance in P123H βS tg mice compared with non-tg littermates (NonTg) at different ages. Data are shown as mean±s.e.m. (n=8–10). *P<0.05, **P<0.01 versus non-tg mice. Figure 3: Behavioural abnormalities of P123H βS tg mice. ( a – c ) The Morris water maze test. Compared with non-tg littermates (NonTg), P123H βS tg mice (lines B and C) at 6 months (mo) did not show an improvement in performance during the training session ( a ). After removing the platform, a probe test was performed on the last day of the training session ( b , c ). P123H βS tg mice spent less time searching in the target quadrant than did non-Tg (N) mice ( b ). Similarly, P123H βS tg mice had less frequency of crossing the goal ( c ). Data are shown as the mean±s.e.m. ( n =7–11). * P <0.05, ** P <0.01 versus non-tg mice. ( d ) Home cage test showing decreased spontaneous activities in P123H βS tg mice (line C) compared with non-tg littermates at 6 months. Time spent in various types of behaviours, including 'Pause' 'Sleep' 'Twitch', 'Groom', 'Sniff', 'Rear up' and 'Hang Vertically', was measured using a video tracking system. 'Awaken' is the end of sleep during this period. Data are shown as mean±s.e.m. ( n =7). * P <0.05, ** P <0.01 versus non-tg mice. ( e ) The rotarod treadmill test showing impaired motor performance in P123H βS tg mice compared with non-tg littermates (NonTg) at different ages. Data are shown as mean±s.e.m. ( n =8–10). * P <0.05, ** P <0.01 versus non-tg mice. Full size image Neuropathology of P123H βS tg mice is not affected by deletion of αS The analysis of P123H βS tg mice unambiguously shows that P123H βS is pathogenic in mouse brain. However, it is unclear whether endogenous murine αS has any role in the neuropathology of P123H βS tg mice. This important question was addressed by a cross-breeding experiment of P123H βS tg with αS KO mice ( Supplementary Methods ), in which various neurodegeneration phenotypes, including neuritic pathology ( Supplementary Fig. S4a ), formation of globular axonal swelling ( Supplementary Fig. S4b ), protein aggregation ( Supplementary Fig. S4c ) and astrogliosis ( Supplementary Fig. S4d,e ), were compared. The results showed that none of these neurodegenerative features were significantly different between P123H βS and P123H βS/αS KO tg mice, indicating that endogenous αS may not be necessarily required for the neuropathology of P123H βS. Enhanced neuropathology in P123H βS/αS double tg mice Next, a further cross-breeding experiment of P123H βS tg with αS-overexpressing tg mice was conducted to assess the combined effects of P123H βS and pathogenic αS on neurodegeneration ( Supplementary Methods ). The neuropathological characterization of Thy-1 promoter-driven αS-expressing tg mice was previously reported [22] , indicating that overexpressed αS is pathogenic in mouse brain. As we expected, bigenic mice overexpressing P123H βS and αS showed an enhanced neurodegenerative phenotype compared with each monogenic tg mouse. Besides lower body weight and high mortality ( Supplementary Fig. S5a,b ), bigenic mouse brains were characterized by increased protein aggregation, as demonstrated by the increased level of both αS and P123H βS in FA fractions ( Supplementary Fig. S5c ). Furthermore, expression of synapse proteins, such as VAMP2, SNAP25 and PSD95, was decreased in bigenic mice compared with littermates ( Supplementary Fig. S5d ). Moreover, various pro-inflammatory factors, including interleukin 1β (IL-1β), IL-6, tumour necrosis factor-α, induced nitrogen oxide synthase and monocyte chemotactic protein-1, were significantly upregulated in bigenic mice compared with littermates, suggesting that neuroinflammation was enhanced in bigenic mice ( Supplementary Fig. S6a ). Indeed, morphologically activated astrocytes and microglia were occasionally observed in bigenic mice but not in littermates ( Supplementary Fig. S6b,c ). Because IL-1β colocalized well with GFAP but not with CD11b, it was predicted that astrocytes may have a dominant role in inflammation in this stage ( Supplementary Fig. S6d,e ). During the terminal stage ( ∼ 9 months) of bigenic mice, numerous phospho-c-Jun- and c-Fos-positive nuclei were observed in the hippocampus and cortex, suggesting that neurons in bigenic mice are subjected to chronic stress ( Fig. 4a,b ). Concordant with these findings, Fluoro Jade C (FJC)-positive degenerating neurons were occasionally observed in bigenic mice and to a lesser extent in αS tg mice ( Fig. 4c ). Given the immunoreactivity of αS in FJC-positive neurons, accumulated αS might directly and continuously injure neurons, leading to stimulation of neurodegeneration ( Fig. 4c ). Such a chronic process of neurodegeneration may eventually lead to neuronal loss, as the numbers of NeuN-immunopositive neurons in the hippocampus of bigenic mice were significantly lower than those of monogenic tg mice and of non-tg littermates ( Fig. 4d ). Nevertheless, terminal deoxynucleotidyl transferase dUTP nick end labelling (TUNEL)-positive neurons were not convincingly detected ( Fig. 4e ), suggesting that non-apoptotic neuronal cell death may at least partly contribute to neuronal loss in bigenic mice. Similar TUNEL-negative neuronal death has been documented in various types of neurodegeneration, including degeneration of dopaminergic neurons induced by 6-hydroxydopamine, axotomy and 1-methyl-4-phenyl-1,2,3,6-tetrahydropyridine (MPTP) in adult mice [23] , [24] . Finally, EM studies consistently demonstrated the presence of degenerating dark neurons in the hippocampus and cortex of bigenic brains, but not in littermates ( Fig. 4f ). Although the mechanism is unknown, dark neurons are induced under a variety of pathological conditions, including ischaemia, epilepsy and head injury [25] . Furthermore, dark neurons have been described in a mouse model and in the brain of a patient affected by Huntington's disease [26] , as well as in an αS-conditioned mouse model of PD [27] and in a MPTP-treated mouse model of PD [28] . Considering that conventional αS tg mice rarely exhibit neuronal death, our bigenic mice may be a powerful tool with which to investigate the mechanism of neuronal death in neurodegenerative diseases. 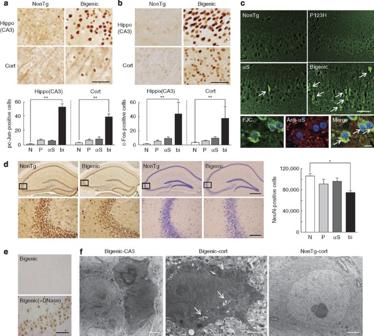Figure 4: Non-apoptotic neurodegeneration in bigenic mice overexpressing P123H βS and αS. Hippocampus (hippo) CA3 and cortex (cort) of 9-month-old bigenic mice and littermates (P123H βS tg, αS tg and non-tg) were analysed. Abbreviations used in graph panels are non-tg, N; P123H βS tg, P; αS tg, αS; and bigenic, bi. (a,b) Immunohistochemistry of pc-Jun (a) and c-Fos (b). Representative images of bigenic mice and NonTg littermates are shown. Scale bar=50 μm. The graph shows quantification of the pc-Jun-positive cell count in 180×180 μm2areas. Data are shown as mean±s.e.m. (n=5 fora,n=8 forb). **P<0.01 versus non-tg mice. (c) Evaluation of neurodegeneration by FJC staining. Representative images of the hippocampus from bigenic mice and from other littermates are shown (four figures in the upper panel). FJC-positive cells were observed in bigenic mice and to a lesser extent in αS tg mice (arrows). Scale bar=50 μm. Lower images show that FJC-stained cells were also positive for αS (arrows) in bigenic mice. Nuclei were simultaneously stained with DAPI (4,6-diamidino-2-phenylindole). Scale bar=10 μm. (d) Immunohistochemistry of NeuN. Representative images of NeuN (four panels to the left) and crystal violet staining (four panels to the right) of the hippocampus from bigenic mice and NonTg littermates are shown. Scale bar=500 μm (upper two panels) or 100 μm (lower two panels). The figures given in the lower panels are magnifications of the figures given in the upper panel. The graph shows neuronal density based on the NeuN-immunoreactive cell count (cells mm−3) in the hippocampus. Data are shown as mean±s.e.m. (n=5). *P<0.05 versus non-tg mice. (e) TUNEL staining. The hippocampus sections from bigenic mice were treated without (upper panel) or with DNase I (lower panel) (n=5). Representative figures are shown. Scale bar=50 μm. (f) Appearance of dark degenerating neurons in the hippocampus and cortex of bigenic mice, but not in NonTg brains, in EM. Neuronal soma and dendritic processes both showed darkened features. Arrows indicate dilated Golgi apparatus in the shrunken cytoplasm (centre). In some cases, membrane structures of the nucleus and cytoplasm were obscure (left), which may reflect the terminal stage of neurodegeneration. Scale bar=2 μm. Figure 4: Non-apoptotic neurodegeneration in bigenic mice overexpressing P123H βS and αS. Hippocampus (hippo) CA3 and cortex (cort) of 9-month-old bigenic mice and littermates (P123H βS tg, αS tg and non-tg) were analysed. Abbreviations used in graph panels are non-tg, N; P123H βS tg, P; αS tg, αS; and bigenic, bi. ( a , b ) Immunohistochemistry of pc-Jun ( a ) and c-Fos ( b ). Representative images of bigenic mice and NonTg littermates are shown. Scale bar=50 μm. The graph shows quantification of the pc-Jun-positive cell count in 180×180 μm 2 areas. Data are shown as mean±s.e.m. ( n =5 for a , n =8 for b ). ** P <0.01 versus non-tg mice. ( c ) Evaluation of neurodegeneration by FJC staining. Representative images of the hippocampus from bigenic mice and from other littermates are shown (four figures in the upper panel). FJC-positive cells were observed in bigenic mice and to a lesser extent in αS tg mice (arrows). Scale bar=50 μm. Lower images show that FJC-stained cells were also positive for αS (arrows) in bigenic mice. Nuclei were simultaneously stained with DAPI (4,6-diamidino-2-phenylindole). Scale bar=10 μm. ( d ) Immunohistochemistry of NeuN. Representative images of NeuN (four panels to the left) and crystal violet staining (four panels to the right) of the hippocampus from bigenic mice and NonTg littermates are shown. Scale bar=500 μm (upper two panels) or 100 μm (lower two panels). The figures given in the lower panels are magnifications of the figures given in the upper panel. The graph shows neuronal density based on the NeuN-immunoreactive cell count (cells mm −3 ) in the hippocampus. Data are shown as mean±s.e.m. ( n =5). * P <0.05 versus non-tg mice. ( e ) TUNEL staining. The hippocampus sections from bigenic mice were treated without (upper panel) or with DNase I (lower panel) ( n =5). Representative figures are shown. Scale bar=50 μm. ( f ) Appearance of dark degenerating neurons in the hippocampus and cortex of bigenic mice, but not in NonTg brains, in EM. Neuronal soma and dendritic processes both showed darkened features. Arrows indicate dilated Golgi apparatus in the shrunken cytoplasm (centre). In some cases, membrane structures of the nucleus and cytoplasm were obscure (left), which may reflect the terminal stage of neurodegeneration. Scale bar=2 μm. Full size image Finally, several findings suggested that dopaminergic dysfunction might be involved in motor dysfunctions of bigenic mice during the middle stage (4–7 months). First, strong clasping was observed in bigenic mice but not in other littermates ( Fig. 5a ). Clasping behaviour has never been observed in C57BL/6 mice during this stage in routine experiments. Furthermore, clasping has been described in various models of nigrostriatal anomalies [29] , [30] . Second, locomotor performance was significantly impaired in bigenic mice compared with αS tg mice and other littermates ( Fig. 5b ). Third, the levels of tyrosine hydroxylase (TH) and other dopaminergic markers, including L -dopa decarboxylase and dopamine transporter, were significantly decreased in the basal ganglia ( Fig. 5c,d ), although it was unclear whether the motor deficits were entirely attributable to the modest decrease ( ∼ 40%) in the dopamine concentration ( Fig. 5e ). In addition, the number of globules in basal ganglia was significantly higher in bigenic mice compared with P123H βS mice ( Supplementary Fig. S7 ). One may speculate that globule formation of GABAergic projection neurons was stimulated by the compensatory mechanism in response to decreased dopaminergic inputs in bigenic mice. Taken together, these results suggest that motor deficits of bigenic mice are attributed to axonal degeneration of nigrostriatal dopaminergic neurons. 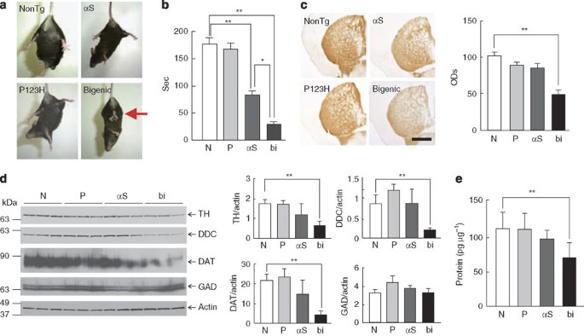Figure 5: Dopaminergic dysfunction in the striatum of bigenic mice. (a,b) Evaluation of the motor functions of bigenic (bi) mice and littermates (αS tg, αS; P123H βS tg, P; and non-tg, N) at 4 months. Ina, a representative photograph of the tail-suspension assay shows strong front and hind limb clasping in bigenic mice (arrow), but not in other littermates. Inb, the rotarod treadmill test shows impaired motor performance in bigenic mice and to a lesser extent in αS tg mice. Data are shown as mean±s.e.m. (n=9–18). *P<0.05, **P<0.01. (c–e) Striata from 7-month-old bigenic mice and littermates (P123H βS tg, αS tg and non-tg) were analysed. Abbreviations used in graph panels are non-tg, N; P123H βS tg, P; αS tg, αS; and bigenic, bi. Inc, representative images of TH immunohistochemistry are shown. Scale bar=500 μm. The average optical densities (ODs) of the TH immunoreactivity was measured. Data are shown as mean±s.e.m. (n=8). **P<0.01 versus non-tg mice. Ind, representative immunoblots of dopaminergic proteins (TH,L-dopa decarboxylase (DDC) and dopamine transporter (DAT)) and glutamic acid decarboxylase (GAD) and quantification of data against actin bands are shown. Data are shown as mean±s.e.m. (n=8). **P<0.01. Ine, dopamine concentrations in the striatum were measured by enzyme-linked immunosorbent assay. Data are shown as mean±s.e.m. (n=5). **P<0.01 versus non-tg mice. Figure 5: Dopaminergic dysfunction in the striatum of bigenic mice. ( a , b ) Evaluation of the motor functions of bigenic (bi) mice and littermates (αS tg, αS; P123H βS tg, P; and non-tg, N) at 4 months. In a , a representative photograph of the tail-suspension assay shows strong front and hind limb clasping in bigenic mice (arrow), but not in other littermates. In b , the rotarod treadmill test shows impaired motor performance in bigenic mice and to a lesser extent in αS tg mice. Data are shown as mean±s.e.m. ( n =9–18). * P <0.05, ** P <0.01. ( c – e ) Striata from 7-month-old bigenic mice and littermates (P123H βS tg, αS tg and non-tg) were analysed. Abbreviations used in graph panels are non-tg, N; P123H βS tg, P; αS tg, αS; and bigenic, bi. In c , representative images of TH immunohistochemistry are shown. Scale bar=500 μm. The average optical densities (ODs) of the TH immunoreactivity was measured. Data are shown as mean±s.e.m. ( n =8). ** P <0.01 versus non-tg mice. In d , representative immunoblots of dopaminergic proteins (TH, L -dopa decarboxylase (DDC) and dopamine transporter (DAT)) and glutamic acid decarboxylase (GAD) and quantification of data against actin bands are shown. Data are shown as mean±s.e.m. ( n =8). ** P <0.01. In e , dopamine concentrations in the striatum were measured by enzyme-linked immunosorbent assay. Data are shown as mean±s.e.m. ( n =5). ** P <0.01 versus non-tg mice. Full size image This study demonstrates that P123H βS is itself pathogenic, and endogenous murine αS is dispensable to the neuropathology of P123H βS tg mice. On the other hand, bigenic mice overexpressing P123H βS and human αS exhibited enhanced neuropathology. These results strongly suggest that P123H βS may cooperate with the pathogenic (overexpressed) state of αS, but not with normal αS, to stimulate neurodegeneration. In this context, it is possible that aggregation of αS in the P123H βS brains of patients might be stimulated not only by P123H βS but also by other factors, such as ageing, genetic factors and environmental risks. Such a notion is in line with the incomplete dominant inheritance in a familial DLB associated with P123H βS mutation and could partly explain Lewy body pathology in the postmortem brain of the patient [14] . It is also intriguing that the present results are in contrast to previous studies showing that neuropathological features of αS tg mice were ameliorated in bigenic mice overexpressing αS and wt βS [7] , [8] . Collectively, one possible interpretation is that the neuroprotective βS might be converted to a neurotoxic molecule by the P123H mutation, leading to stimulation of αS pathology. The precise mechanism of neurotoxic conversion of βS by the P123H mutation is currently unknown. In this regard, it is of note that the C-terminal region of βS is composed of a polyproline II helix, unfolding of which may have an important role in protein–protein interactions [31] . Thus, the P123H substitution may affect the polyproline II helix structure, resulting in a conformational change and misfolding of βS that leads to stimulation of αS oligomerization. Because the C-terminal region of βS is subjected to post-translational modification through phosphorylation [1] and glycosylation [32] , it is also possible that aberrant regulation of the C-terminal region by various stimuli may contribute to the involvement of βS in sporadic cases of α-synucleinopathies. Indeed, the neuritic pathology of P123H βS mice is reminiscent of previous reports showing that βS and γ-synuclein (γS), the third member of the synuclein family of peptides, are associated with neuritic pathology, such as in dystrophic neurites and spheroid structures, in the brains of sporadic cases of PD, DLB and neurodegeneration with brain iron accumulation, type 1 [33] , [34] . Our findings and a recent report showing that overexpression of γS results in neurodegeneration in mouse brain [35] indicate the need for future studies to determine whether altered βS and possibly γS may cooperate with αS in the pathogenesis of a broad range of α-synucleinopathies. Summary of the generation and analysis of tg mice All animal procedures were approved and conducted in accordance with Animal Ethics Review Committee regulations of the Tokyo Metropolitan Institute for Neuroscience. For generation of tg mice expressing P123H βS, human P123H βS cDNA was released from a PCEP4-P123H βS vector [15] and inserted into the Xho I site of the mouse Thy-1 expression cassette (kindly supplied by Dr H van der Putten, Ciba-Geigy). The Thy-1-P123H βS plasmids were microinjected into fertilized eggs of C57BL/6 mouse and multiple lines of Thy-1-P123H βS tg mice were generated. Thy1-αS tg mice and Thy1-wt βS tg mice were both primarily established as DBA2 × C57BL/6 hybrids [7] , [22] . These mice were maintained by successive (more than seven generations) backcrossing into the C57BL/6 strain. Heterozygote Thy1-P123H βS tg mice (line C: the highest expresser) were further crossed with heterozygote Thy1-αS tg mice to generate bigenic mice overexpressing human P123H βS and human αS, and littermates including P123H βS tg mice, αS tg mice and non-tg mice. Genomic DNA was extracted from tail biopsies, and genotyping of P123H βS and human αS was performed by PCR using specific primers ( Supplementary Table S1 ). The tg mice were evaluated by histological and biochemical analyses using various antibodies ( Supplementary Methods , Supplementary Table S2 ), in addition to several behavioural tests. Tissue processing of tg mice brain Mice brains were removed under deep anaesthesia and divided sagittally. One hemibrain was snap frozen in liquid nitrogen and stored at −80 °C for biochemical studies and RNA analysis. Hippocampus and cortex samples were collected from the region 1.8–2.8 mm posterior to the bregma, whereas striatum samples were obtained from the region 0–1 mm anterior to the bregma. The other hemibrain was fixed in Bouin's solution and embedded in paraffin for preparation of 4 μm serial sections for analysis. Free-floating brain sections were prepared by transcardiac perfusion with ice-cold saline, followed by 4% paraformaldehyde or Zamboni's solution containing glutaraldehyde. Serial sections of 40-μm thickness were then prepared. For the hippocampus and cortex, sagittal sections ∼ 1.5 mm lateral to the midline or coronal sections ∼ 1.5 mm posterior to the bregma, were used. For the striatum and globus pallidus, sagittal sections ∼ 1.5 mm lateral to the midline or coronal sections ∼ 0.5 mm anterior to the bregma were used. For the substantia nigra, coronal sections ∼ 2.6 mm posterior to the bregma were used. The location of the slice and identification of brain regions were determined by comparison to atlas images [36] . Northern blot analysis Total RNA isolated from whole brains was analysed by northern blotting, as previously described [37] . Hybridization was performed using 32 P-P123H βS cDNA labelled by random priming. The filter was reprobed with 32 P-labelled actin cDNA. The intensities of the hybridization bands were measured using BioMAX 1D image analysis software (Kodak). Immunoblot analysis Mice brains were homogenized in lysis buffer containing 1% Triton X-100 [38] and centrifuged at 100,000 g for 30 min. The supernatants (10 μg) were resolved by SDS–PAGE and electroblotted onto nitrocellulose membranes. The membranes were blocked with 3% bovine serum albumin in Tris-buffered saline (TBS) plus 0.2% Tween 20, followed by incubation with primary antibodies in TBS containing 3% bovine serum albumin. After washing, the membranes were further incubated with secondary antibody conjugated with horseradish peroxidase in TBS (1:5,000 ∼ 10,000). Finally, the target proteins were visualized with the ECL plus system (GE Healthcare), followed by quantification using BioMAX 1D image analysis software. Immunohistochemistry and immunofluorescence Immunohistochemistry was performed as previously described [7] . Briefly, paraffin sections were autoclaved in 0.01 M citrate buffer (pH 6.0) to retrieve antigen. Both paraffin and free-floating sections were then immersed in 0.3% hydrogen peroxide in methanol and incubated in 5% normal goat or rabbit serum for blocking. Sections were incubated with primary antibodies overnight at 4 °C, followed by detection with biotinylated secondary antibodies and the Avidin–Biotin Complex Kit (Vector Laboratories). A positive reaction was detected using diaminobenzidine tetrahydrochloride containing 0.001% hydrogen peroxide. The results from at least seven images of serial sections for each mouse were used and an average value was calculated. Cells were counted and optical densities were measured in some immunohistochemistry experiments. Stereological analysis was conducted with MCID image analysis software (InterFocus Imaging) for NeuN-immunoreactive cells in the hippocampal CA3 region and cerebral cortex and for TH-immunoreactive cells in the substantia nigra, as previously reported [39] , [40] . In brief, digital images of NeuN- and TH-immunoreactive neurons were acquired at ×50 magnification on an Olympus microscope fitted with a video camera (Olympus). A counting frame created by the MCID image analysis software was systemically passed over the outlined CA3, cerebral cortex areas and substantia nigra pars compacta. The neurons were counted as they appeared within the counting frame. The average neuron density was obtained by totalling the number of neuron profiles and dividing by the calculated area [41] , [42] . As for P123H βS-immunoreactive cells in the globus pallidus, positive cells with a diameter of >3 μm were selectively counted. For phospho-c-Jun- and c-Fos-immunoreactive cells, counting was conducted in areas of 180×180 μm 2 in the hippocampus and cortex. For TH-immunoreactive fibres in the striatum, the average optical densities were evaluated as previously reported [40] . Immunofluorescence was performed as previously described [7] . Both paraffin and free-floating sections were incubated with primary antibodies, followed by Alexa Fluor-conjugated secondary antibodies (Invitrogen). FJC staining was performed according to the manufacturer's instructions (Chemicon). Slides were observed by laser scanning confocal microscopy [7] . Electron microscopy EM was performed as previously described with modifications [15] . The mice were deeply anaesthetized and killed by cardiac perfusion using ice-cold saline, followed by 2% paraformaldehyde and 2% glutaraldehyde. Brain tissues were post-fixed with 1% osmium tetroxide, followed by dehydration and embedding in Quetol 812 (Nisshin EM). Ultrathin sections were cut, stained with uranyl acetate and lead nitrate and observed using a Hitachi H-7650 electron microscope (Hitachi) equipped with a CanoScan 9900F digital imaging system (Canon). Behaviour tests Learning and memory were analysed with a Morris water maze test, as previously described, with modifications [43] . A circular pool (diameter 1.5 m, height 30 cm, temperature 23±1 °C) was filled with water containing non-fat dry milk. The escape platform (diameter 10 cm) was located in the centre of one of the quadrants of the pool. To habituate mice to the water, the mice were pre-trained 1 day before starting the training session. Each mouse was placed on the visible platform, forced to jump into the water, allowed to swim for 60 s and then guided to the escape platform. This procedure was repeated twice for each mouse. During the training session, mice were trained to find the platform submerged 1 cm below the water surface. If the mouse failed to find the platform within 60 s, it was guided to the platform and allowed to remain there for 15 s. Mice received two trials per day and were trained for 10 days. On the last day of training, the probe test was performed to measure the searching behaviour in the target quadrant (quadrant where the platform was located during training) and platform area (the area where the platform was located) for 60 s. A video tracking system (Topscan; Clever System) was used to analyse the escape latency and swim path. To evaluate the spontaneous behaviour of mice, a home cage test was performed as previously described [44] with modifications. One day before starting the test, mice were isolated and put into the test cage. A paper sheet was used as bedding material instead of sawdust for this test to prevent mice hiding in sawdust during recording. The recorded video during the dark phase (1900–0700 hours) was analysed using Home cage scan software (Clever System). The behavioural definitions, including 'Pause', 'Sleep', 'Twitch', 'Awaken', 'Groom', 'Sniff', 'Rear up' and 'Hang Vertically', are described elsewhere [44] . To measure locomotor activity, the rotarod test was performed as previously described [7] . Briefly, on the first day, mice were trained for three trials: the first one at 5 r.p.m., the second at 10 r.p.m. and the third at 20 r.p.m. On the second day, mice were tested for seven trials. Mice were placed individually on the rod and the speed of rotation was increased from 0 to 40 r.p.m. over 240 s. The length of time mice remained on the rod was recorded and the last four trials were averaged as a measure of motor function. TUNEL assay TUNEL staining was performed using the In Situ Cell Death Detection Kit POD (Roche) according to the manufacturer's instructions. For a positive control, the section was incubated with 10 U ml −1 DNase I (Sigma) for 10 min at room temperature. Dopamine enzyme-linked immunosorbent assay Dopamine concentrations were measured using a Dopamine Research ELISA Kit according to the manufacturer's instructions (Labor Diagnostika). Statistics Data are presented as mean±s.e.m. Statistical differences were determined by either two-tailed t -test or analysis of variance, followed by a post-Fisher's protected least significant difference test, with P <0.05 considered to indicate a significant difference. How to cite this article: Fujita, M. et al . A β-synuclein mutation linked to dementia produces neurodegeneration when expressed in mouse brain. Nat. Commun. 1:110 doi: 10.1038/ncomms1101 (2010).